Stereoselectivity control in Rh-catalyzedβ-OH elimination for chiral allene formation Stereoselectivity control and understanding in the metal-catalyzed reactions are fundamental issues in catalysis. Here we report sterically controlled rhodium-catalyzed S N 2’-type substitution reactions of optically active tertiary propargylic alcohols with arylmetallic species affording the non-readily available enantioenriched tetrasubstituted allenes via either exclusive syn - or anti - β -OH elimination, respectively, under two sets of different reaction parameters. Detailed mechanistic experiments and density functional theory (DFT) studies reveal that the exclusive anti -Rh(I)-OH elimination is dictated by the simultaneous aid of in situ generated boric acid and ambient water, which act as the shuttle in the hydroxy relay to facilitate the Rh(I)-OH elimination process via a unique ten-membered cyclic transition state ( anti - TS2_u ). By contrast, the syn -Rh(III)-OH elimination in C–H bond activation-based allenylation reaction is controlled by a four-membered cyclic transition state ( syn- TS3 ) due to the steric surroundings around the Rh(III) center preventing the approach of the other assisting molecules. Under the guidance of these mechanistic understandings, a stereodivergent protocol to construct the enantiomer of optically active tetrasubstituted allenes from the same starting materials is successfully developed. Stereoselectivity control is an ever-lasting topic in synthesis. Transition metal-catalyzed asymmetric coupling reaction is one of the most powerful tools to construct optically active allenes [1] , [2] , [3] . Stereoselective β -elimination of vinylic metallic species has become one of the most common approaches for asymmetric allene syntheses: In 2013, Frantz and coworkers reported an elegant Pd-catalyzed enantioselective vinyl triflate-based β -H elimination reaction to prepare chiral 1,3-disubstituted allenes (Fig. 1a ) [4] . Recently, Zhang’s group and our group have jointly demonstrated a Pd-catalyzed asymmetric Heck reaction between aryl triflates and internal alkynes to furnish chiral trisubstituted allenes in good yields with high ees via β -H elimination (Fig. 1b ) [5] . The chiral allene formation reactions catalyzed by palladium occur via a well-known syn -elimination mechanism; however, a comprehensive understanding of the stereoselectivity in rhodium catalyzed reactions, specifically the β -OH elimination step, remains unexplored. To the best of our knowledge, the rhodium-catalyzed anti - β -OH elimination has not been reported, therefore, the studies on this elementary reaction process are of fundamental interest. Herein, we wish to report the steric control in rhodium-catalyzed S N 2’-type substitution reaction between optically active tertiary propargylic alcohols and arylmetallic species affording enantioenriched tetrasubstituted allenes [6] , [7] , [8] , [9] , [10] , [11] , [12] , [13] , [14] , [15] , [16] , [17] , [18] , [19] , [20] , [21] , [22] , [23] , [24] , [25] , [26] , [27] , [28] , [29] , [30] , [31] , [32] , [33] , [34] , [35] , [36] , [37] , [38] , [39] , [40] , [41] , [42] under two sets of different reaction conditions (Fig. 1c ). We believe that such understanding on steric control of β -OH elimination provides a new perspective to the stereoselectivity control in metal-catalyzed allene formation reactions. Fig. 1: Metal-catalyzed stereoselective β -elimination processes for syntheses of chiral allenes. a Enantioselective vinyl triflate-based β -H elimination. b Enantioselective alkyne-based β -H elimination. c Steric control on β -OH elimination: syn - vs anti -. Full size image We began our study on the reaction of ( S )-2-phenyloct-3-yn-2-ol ( S )- 1a of ≥99% ee with phenylboronic acid 2a in the presence of different rhodium catalysts with 1,4-dioxane as the solvent. 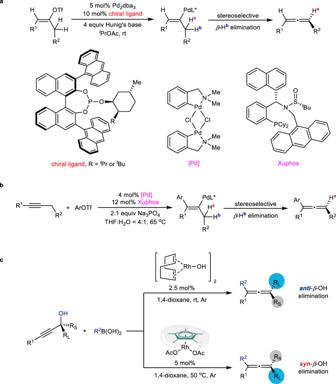Fig. 1: Metal-catalyzed stereoselectiveβ-elimination processes for syntheses of chiral allenes. aEnantioselective vinyl triflate-basedβ-H elimination.bEnantioselective alkyne-basedβ-H elimination.cSteric control onβ-OH elimination:syn- vsanti-. [Cp*RhCl 2 ] 2 and Rh 2 (OAc) 4 failed to afford the desired tetrasubstituted allene product 3aa with 98-99% recovery of ( S )- 1a (Table 1 , entries 1−2). Interestingly, 65% yield of ( R )- 3aa with 93% ee was obtained when [Rh(COD)Cl] 2 was applied as the catalyst (Table 1 , entry 3). Then different Rh(I) catalysts were examined for the reactions in 1,4-dioxane (Table 1 , entries 4−8) and [Rh(COD)OH] 2 turned out to be best, affording ( R )- 3aa in 89% yield and 97% ee at 50 ° C (Table 1 , entry 8). The absolute configuration of optically active 3aa was tentatively assigned to be R based on the Lowe-Brewster rule [43] , [44] . The solvent effect was further studied. Ethers, such as THF, DME, Et 2 O, and MTBE, are also suitable solvents for this transformation, which afforded ( R )- 3aa in 81−87% yields with no less than 91% ees (Table 1 , entries 10−13). Ethyl acetate or even acetone could afford ( R )- 3aa in 99% or 97% ee (Table 1 , entries 14 and 15). Interestingly, even MeOH could afford ( R )- 3aa with 93% ee (Table 1 , entry 16). When DCM, DCE, toluene, or DMF was used as the solvent, ( R )- 3aa was obtained in diminished yields (Table 1 , entries 17−20). 100% of ( S )- 1a was recovered when the reaction was conducted in MeCN (Table 1 , entry 21, for more details on the solvent effect, see: page S50 in the Supplementary Information). Furthermore, 94% yield of ( R )- 3aa was obtained with 98% ee when 2.5 mol% of the rhodium catalyst was applied (Table 1 , entry 22). Thus, the optimal reaction conditions for the exclusive anti - β -OH elimination [45] , [46] have been identified as shown in entry 22 of Table 1 , which have been defined as standard Conditions A. Table 1 Optimization of reaction conditions Full size table Mechanistic studies In order to firmly establish the steric outcome of this reaction, ( S )- 1a was converted to its 3,4,5-trimethoxybenzoate ( S )- 1a’ . The absolute configurations of propargylic alcohol ( S )- 1a and the corresponding allene product ( R )- 3ad were then determined via the single crystal X-ray crystallography of ( S )- 1a’ and ( R )- 3ad (Fig. 2a ). With the purpose of further confirming the steric outcome, ( S )- 1j with a heavy atom of bromine was applied (Fig. 2b ). The X-ray diffraction studies of solid aldehyde ( S )- 1j’ and the corresponding product ( R )- 3jd double confirmed the exclusive anti -Rh-OH elimination process. Fig. 2: Establishment of the stereochemical outcome. a X-ray diffraction studies of ( S )- 1a’ and ( R )- 3ad . b X-ray diffraction studies of ( S )- 1j’ and ( R )- 3jd with bromine. The hydrogen atoms are omitted for clarity. Full size image A series of designed experiments were conducted to get insight into the nature of this reaction: The reaction of ( S )-2,4-diphenylbut-3-yn-2-ol ( S )- 1b (91% ee) furnished the target product ( R )- 3bb in 50% yield with 90% ee and 43% yield of the hydroarylation product ( R , E )- 4bb with 90% ee (Fig. 3a ). This result indicated that an alkenylrhodium int. A was formed via a regioselective syn -insertion of the C-C triple bond into the aryl-rhodium bond formed by the transmetalation of rhodium hydroxide species with arylboronic acid. Fig. 3: Mechanistic studies. a The reaction of ( S )- 1b with aryl boronic acid 2b . b The reaction of ( S )- 1a with different boron reagents. c Monitoring experiment via 11 B NMR. d The role of H 2 O. e Further investigation on the effect of H 2 O by using dried starting materials and solvent with the deliberate addition of water. Full size image When other boron reagent, such as (PhBO) 3 , PhBF 3 K, PhBneop, or PhBpin, was submitted to the standard Conditions A, only triphenylboroxin afforded the desired product in 92% yield with 99% ee (Fig. 3b ). In the presence of propargylic alcohol and ambient water, triphenylboroxin may undergo hydrolysis to form phenylboronic acid. These results suggested that boric acid, which was formed after transmetalation, may involve in the reaction and play a critical role. To confirm this hypothesis, the reaction of ( S )- 1a with arylboronic acid 2c in the THF- d 8 was monitored by 11 B NMR experiment and the signal of B(OH) 3 ( δ = 20.1 ppm) was observed (Fig. 3c ). To unveil the effect of ambient water in this reaction, several control experiments were performed. The reaction in the presence of 1.0 equiv of H 2 O afforded an even slightly better result (95% yield, 96% ee, >99% es) as compared to the result under the standard conditions (Fig. 3d , entry 1 vs entry 2). When 20 mg of 4 Å molecular sieve were submitted to the reaction, the target product ( R )- 3aa was obtained in 63% yield with 91% ee (Fig. 3d , entry 3). Based on these results, the starting materials (( S )- 1a and organoboron 2a ) and 1,4-dioxane were carefully dried (for full details, see: pages S49−50 in Supplementary Information) to further explore the effect of H 2 O on the Rh- β -OH elimination process. The reactions proceeded smoothly via an exclusive anti -OH elimination process in the presence of a specific amount of H 2 O, forming ( R )- 3aa in very high yields (Fig. 3e , entries 1-3). There was no significant change when PhB(OH) 2 or (PhBO) 3 was applied (Fig. 3e , entries 4 and 5). However, compared to the results under the standard conditions (Fig. 3e , entry 4 vs Fig. 3d , entry 2), a slight influence on the ee value was observed (93% ee vs 95% ee). Much lower ee for allene product ( R )- 3aa was observed by running the reaction in the presence of 20 mg or 40 mg of 4 Å molecular sieve (Fig. 3e , entries 6 and 7). All these results indicated that the ambient water may play a critical role on the stereoselectivity of this Rh-OH elimination reaction. To shed light on the unique nature of anti -OH elimination, detailed density functional theory (DFT) calculations were carried out by using ( S )-2-phenylpent-3-yn-2-ol ( S )- 1A as the model (for details of the computational methods, see: page S75 in the Supplementary Information and calculated coordinates of the optimized structures in Supplementary Data 1 ). The formation of complex Int1 , which was selected as the free energy reference, involves the coordination of the triple bond in ( S )- 1A with the rhodium atom in metallic species I (Fig. 4a ). The syn -insertion proceeds irreversibly via transition state TS1 with a free energy barrier of only 6.0 kcal/mol resulting in the formation of the intermediate Int2 . The subsequent direct syn-β -OH elimination via a four-membered ring transition structure syn- TS2 would lead to the formation of the final ( S )-product. However, considering the fact that ( R )-products were obtained via an exclusive anti - β -OH elimination experimentally, there must be other possible pathways. Fig. 4: DFT calculations and proposed mechanism for the reaction of ( S )-2-phenylpent-3-yn-2-ol ( S )-1A with phenyl-rhodium I. a Energy profiles for the syn -insertion and the direct β -OH elimination processes of ( S )- 1A with phenyl-rhodium I (Free energies are given in kcal/mol with respect of Int1 ). b The transition states for B(OH) 3 and H 2 O assisted anti - β -OH elimination process (Bond lengths are given in angstroms). c The proposed mechanism. Full size image Previous control experiments (Fig. 3b–e ) confirmed the critical role of the in situ generated boric acid and ambient water in the reaction. Thus, by utilizing one, two, or three molecules of boric acid or water as the hydroxy shuttle, a series of concerted six-, eight-, or ten-membered cyclic transition structures TS2_a-z were obtained regarding Rh- β -OH elimination (for details, see: Supplementary Figs. 4 – 7 ). Among these transition states, the concerted ten-membered syn - TS2_i and anti - TS2_u , were obtained, respectively, as the most stable syn - and anti - β -OH elimination transition structures (Fig. 4b ). These two transition structures exhibit activation free energy barriers of 9.7 and 7.6 kcal/mol, respectively, which are more favorable than the direct four-membered ring syn - TS2 (Fig. 4a , 19.5 kcal/mol). Notably, both syn - TS2_i and anti - TS2_u involve the collaboration of two molecules of boric acid and one molecule of water. Further examination discovered that the syn- TS2_i experiences a steric repulsion caused by the assisting species B(OH) 3 with COD ligand, exhibiting a minimal H–H bond distance of only 2.27 Å. As a comparison, no apparent steric repulsions have been detected in anti - TS2_u . Moreover, there is also difference of the bond angle of C 1 , C 2 and C 3 , which are 119.9° in syn- TS2_i and 123.5° in anti- TS2_u , respectively (Fig. 4b ). By comparison, the bond angle of C 1 , C 2 and C 3 is 128.9° in their precursor Int2 and 150.4° in the corresponding product Int3 , which indicates that the C 1 , C 2 , and C 3 unit in syn- TS2_i experiences a greater distortion than that in anti - TS2_u (Supplementary Fig. 7 ). Thus, the relative instability of syn- TS2_i compared to anti- TS2_u originates from the steric repulsion between B(OH) 3 and COD ligand as well as the greater distortion of the C 1 , C 2 , and C 3 unit in syn - TS2_i . We, therefore, concluded that the participation of molecules like boric acid and/or water could potentially act as a hydroxy shuttle, aiding in the formation of larger ring transition structures to facilitate the anti - β -OH elimination. Based on the experimental and computational data, a rationale for the reaction has been proposed as shown in Fig. 4c : Transmetalation of Rh–OH with arylboronic acid would form the boric acid and aryl-rhodium intermediate I , which was followed by the regioselective syn -insertion of the C-C triple bond to form the intermediate II [42] . Subsequently, in situ generated boric acid and ambient water facilitated the stereospecific anti - β -OH elimination via concerted ten-membered cyclic transition state anti - TS2_u , leading to the formation of the final product ( R )- 3 . Subsequently, we turned our attention back to investigate the factor governing the unique exclusive syn - β -OH elimination observed in our earlier study on the Rh-catalyzed direct reactions of optically active tertiary propargylic alcohols with N -methoxybenzamides [45] . As mentioned above, the simultaneous participation of boric acid and water may play a crucial role in the anti -Rh-OH elimination pathway. Thus, we carried out the control experiments to investigate the effect of boric acid on the syn - β -OH elimination reaction. Obviously, the reaction of ( S )- 1a still afforded ( S )- 16 in the presence of 1 equiv of boric acid (Fig. 5a , entry 1 vs entry 2). Further DFT calculations were subsequently conducted on the β -OH elimination step from the corresponding rhodacyclic intermediate Int4 (Fig. 5b ), which was generated via the Rh-involved CMD (concerted metalation/deprotonation) process and subsequent regiospecific insertion of the alkyne. In the absence of the assisting molecules, the direct β -OH elimination of Int4 proceeds in syn manner via a four-membered transition structure syn - TS3 (Fig. 5c ), which requires an energy barrier of 14.4 kcal/mol, leading to the formation of the final product ( S )- 17 [45] . We conducted further DFT calculations to investigate the effect of the assisting species, such as water, acetic acid, and boric acid, on the β -OH elimination step. Unfortunately, computational analysis revealed that all transition states TS3_a-g involving the assisting molecules (for details, see: Supplementary Figs. 8 – 10 ) were predicted to be unfavorable when compared to syn - TS3 (Fig. 5c ). This is attributed to the strong coordination of the η 5 -Cp* ligand with the Rh(III) center, creating a very crowded environment preventing the approaching of other assisting molecules. For example, the participation of a boric acid molecule raises the activation energy of the syn - β -OH elimination to 26.6 kcal/mol via syn - TS3_c (Fig. 5c ), characterized by an minimal H–H bond distance of only 2.30 Å. Remarkably, to circumvent steric hindrance, the Cp* ligand would exhibit an unusual η 1 -coordination mode with the Rh(III) center in the anti - TS3_g structure instead of the conventional η 5 -coordination, resulting in the much unfavorable anti - TS3_g with a high energy barrier of 38.1 kcal/mol (Fig. 5c ). Therefore, it is reasonable to conclude that the highly congested surroundings created by the strong coordination of the η 5 -Cp* ligand with the Rh(III) center effectively block the approach of other assisting molecules, thus, making direct syn - β -OH elimination ( syn - TS3 ) the most favorable pathway. Fig. 5: Control experiments and DFT calculations for [Cp*RhCl 2 ] 2 catalyzed reaction of chiral propargylic alcohol ( S )-1B with N -methoxybenzamide [45] . a Control experiments with or without boric acid. b [Cp*RhCl 2 ] 2 catalyzed reaction of chiral propargylic alcohol ( S )- 1B with N -methoxybenzamide affording chiral allene ( S )- 17 via syn - β -OH elimination of Int 4 . c The transition states for syn - or anti - β -OH elimination process (Bond lengths are given in angstroms). Full size image After unveiling the steric hinderance of Cp* ligand around the rhodium center as the possible critical factor for the syn - β -OH elimination process for the reaction of the chiral propargylic alcohols with N -methoxybenzamides [45] , further optimization experiments were performed for realizing the syn - β -OH elimination for the reaction of optically active propargylic alcohols with aryl boronic acids. Indeed, with ( S )-2-phenyloct-3-yn-2-ol ( S )- 1a and phenylboronic acid 2a as the model starting materials, when [Cp*RhCl 2 ] 2 and NaOAc were applied instead of [Rh(COD)OH] 2 , 17% yield of ( S )-allene product, ( S )- 3aa , was formed. 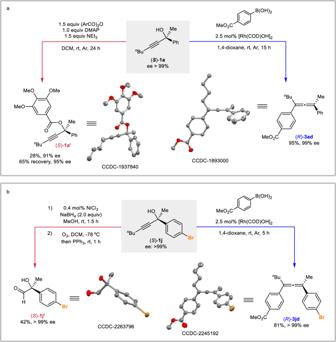Fig. 2: Establishment of the stereochemical outcome. aX-ray diffraction studies of (S)-1a’and (R)-3ad.bX-ray diffraction studies of (S)-1j’and (R)-3jdwith bromine. The hydrogen atoms are omitted for clarity. To further improve the efficiency of this transformation, the reaction parameters including the loading of NaOAc, temperature, and reaction time were further optimized, however, the conversion was still low (Table 2 , entries 2–6). We then turned our attention to the different Cp* ligand containing rhodium catalysts: No desired allene product was observed with Cp*Rh(MeCN) 3 (SbF 6 ) 2 as catalyst (Table 2 , entry 7); interestingly, ( S )- 3aa was obtained in 90% yield with 99% ee by employing the Cp*Rh(OAc) 2 as catalyst. Thus, the second set of optimal reaction conditions for the exclusive syn - β -OH elimination, defined as standard Conditions B, has been established as shown in entry 8 of Table 2 . Table 2 Optimization of reaction conditions for exclusive syn - β -OH elimination Full size table Detailed DFT calculations were then conducted on the Cp*Rh(OAc) 2 -catalyzed syn - β -OH elimination process (Fig. 6 ). The insertion step is computed to be exergonic (ΔG sol = -33.9 kcal/mol) and requires an activation barrier of 11.8 kcal/mol ( TS1’ , Fig. 6a ), leading to the formation of the intermediate Int2’ . 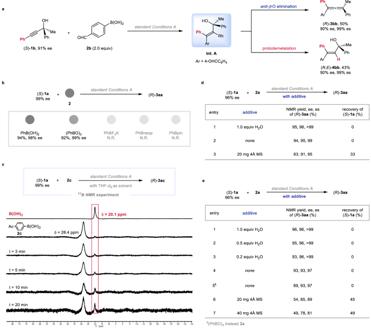Fig. 3: Mechanistic studies. aThe reaction of (S)-1bwith aryl boronic acid2b.bThe reaction of (S)-1awith different boron reagents.cMonitoring experiment via11B NMR.dThe role of H2O.eFurther investigation on the effect of H2O by using dried starting materials and solvent with the deliberate addition of water. Subsequent direct syn - β -OH elimination step would afford ( S )- 3Aa via syn - TS4 requiring a free energy barrier of 26.4 kcal/mol. When the assisting species (water or/and boric acid) are taken into consideration, the syn - β -OH elimination TS s and anti - β -OH elimination TS s are all less favorable as compared with syn - TS4 (for details, see: Supplementary Figs. 11 – 14 ). For instance, one molecule of boric acid destabilized the syn-β- OH elimination by 15.2 kcal/mol ( syn- TS4_b vs. syn- TS4 , Fig. 6b ). A substantial difference is discernible referring to the bond angle of C 1 , C 2 , and C 3 , measuring 119.9° in syn- TS4_b and 134.6° in syn- TS4 , respectively (Fig. 6b ). This remarkable difference suggests that the C 1 , C 2 , and C 3 unit undergoes greater distortion in syn- TS4_b as compared to syn- TS4 (Supplementary Fig. 14 ). Furthermore, anti - TS4_e , exhibiting an abnormal η 1 -coordination mode of the Cp* ligand with Rh(III) center, displayed a relatively high free energy barrier of 47.8 kcal/mol. Thus, the same conclusion can be drown that the strong coordination of the η 5 -Cp* ligand with the Rh(III) center produces a highly congested environment that hinders the approach of other assisting molecules, ultimately resulting in a preference for direct syn - β -OH elimination. Fig. 6: DFT calculations on Cp*Rh(OAc) 2 catalyzed syn-β -OH elimination of ( S )-2-phenylpent-3-yn-2-ol ( S )-1A with Cp*PhRh(III)(OAc) I’. a Energy profiles for reaction of ( S )- 1A with Cp*PhRh(OAc) involving the syn -insertion and syn-β -OH elimination process of Int 2’ (Free energies are given in kcal/mol). b The transition states for syn - or anti - β -OH elimination process (Bond lengths are given in angstroms). Full size image Substrate scope By employing the above optimized conditions (Table 1 , entry 22), the scope of the reaction involving different aryl boronic acids was first explored with ( S )- 1a (Fig. 7 , Condition A). Various electron-withdrawing synthetically versatile functional groups including formyl, acetyl, ester, nitro, trifluoromethyl, and halides were well tolerated in this reaction, affording the desired products ( R )- 3ab − 3ai in 88–97% yields with no less than 95% ee. Introducing the electron-donating groups, such as methoxy and tert -butyl, to the para -position of the phenyl group rendered the reaction to give products ( R )- 3aj and ( R )- 3ak in 80% yield with 96% ee and 94% yield with 97% ee, respectively. Aryl boronic acids with the ortho -, meta -, and para -methyl-substituent in the phenyl moiety afforded the desired products ( R )- 3am − 3ao in high yields (76%–99%) with 95%–96% ees, indicating there is no obvious steric effect. Moreover, 1-naphthylboronic acid also worked smoothly affording ( R )- 3ap . Various tertiary propargylic alcohols were also surveyed under the optimized reaction conditions. R 1 group could be n C 5 H 11 , n C 6 H 13 , -(CH 2 ) 4 Cl, and -(CH 2 ) 2 Ph, affording products ( R )- 3cb , ( R )- 3dh , ( R )- 3ea , ( R )- 3ec , and ( R )- 3fq in gratifying results (90%–97% yields with 90%–95% ees). The substrate containing 3-thienyl group reacted under the standard conditions to give the corresponding product ( R )- 3ga in 93% yield with 87% ee. R 3 may also be an aryl group substituted with different substituents on the 2-, 3-, or 4-position, providing the desired products ( R )- 3hi , ( R )- 3ih , and ( R )- 3jb in good yields with an excellent enantiomeric excess. When R 2 is an Et group, the corresponding product ( R )- 3kh was obtained in 82% yield with 99% ee. On the other hand, using the steric hindered catalyst Cp*Rh(OAc) 2 (conditions B), exclusive syn -elimination process has been achieved: The reaction of phenylboronic acid with ( S )- 1a could give ( S )- 3aa in 82% yield with 99% ee; the reaction is amenable to both the electron-withdrawing groups, such as fluoro, phenyl, and ester, and electron-donating group tert -butyl with the formation of the corresponding enantiomeric allene products ( S )- 3ag - 3ar in 56–73% yields with 99% ees from the same starting materials. Fig. 7: The substrate scope. Conditions A for exclusive anti - β -OH elimination: ( S )- 1 (0.2 mmol), 2 (0.4 mmol), and [Rh(COD)OH] 2 (2.5 mol%) in 1,4-dioxane (1 mL) at rt. Conditions B for exclusive syn - β -OH elimination: ( S )- 1 (0.2 mmol), 2 (0.6 mmol), and Cp*Rh(OAc) 2 (5 mol%) in 1,4-dioxane (1 mL) at 50 ° C. Full size image Synthetic applications To demonstrate the synthetic potentials of this protocol, 1.0101 g of ( S )- 1a and 2.0 equiv of 4-formylphenylboronic acid 2b were subjected to the optimized reaction conditions A to give ( R )- 3ab in 87% yield with 96% ee (Fig. 8a ). The skeletons of bioactive compounds (estrone and lithocolic acid) and drug molecules (indometacin and adapalene) were successfully introduced via the copper-catalyzed enantioselective allenation of their terminal propargylic ethers 5 - 8 (EATA reaction) [15] , [47] with the aldehyde functionality in chiral allene ( R )- 3ab affording a series of bisallene products 9 – 12 , which contain a chiral tetrasubstituted allene unit and a chiral 1,3-disubstituted allene motif in moderate yields with excellent diastereoselectivities (Fig. 8b ). In addition, the 1,2-addition of (trimethylsilyl)ethynyl lithium with this aldehyde entity followed by iron-catalyzed aerobic oxidation reaction [48] afforded alkynyl ketone ( R )- 13 in 74% yield with 97% ee without touching the allene unit (Fig. 8c ). The ester functionality in ( R )- 3ad may be reduced with LiAlH 4 to afford the corresponding alcohol ( R )- 14 in 89% yield without erosion of ee (Fig. 8d ). Allene ( R )- 15 was obtained in 92% yield with 93% ee by Suzuki coupling reaction [49] of ( R )- 3ai with 4-formylphenylboronic acid (Fig. 8e ). Fig. 8: Gram-scale reaction and synthetic transformations of the products. a Gram-scale reaction. b Copper-catalyzed enantioselective allenation of ( R )- 3ab with terminal propargylic ethers 5 – 8 . c Synthesis of alkynyl ketone ( R )- 13 from ( R )- 3ab . d Reduction of ( R )- 3ad to alcohol ( R )- 14 with LiAlH 4 . e Suzuki coupling reaction of ( R )- 3ai to ( R )- 15 with 2b . Full size image In this work, we have demonstrated the Rh(I)-catalyzed exclusive anti-β -OH elimination of an alkenylmetal species forming enantioenriched tetrasubstituted allenes from readily available optically active tertiary propargylic alcohols [50] and arylboronic acids with an excellent efficiency of chirality transfer. Experimental evidences reveal that assisting molecules such as boric acid and water play a critical role on this exclusive anti -Rh(I)-OH elimination process and DFT calculations led to a ten-membered cyclic transition state consisting of [2B(OH) 3 ]-[1H 2 O] with an energy as low as 7.6 kcal/mol. And DFT studies suggest that the previously reported exclusive syn -Rh(III)-OH elimination is controlled by a four-membered cyclic transition state ( syn- TS3 ), due to the steric surroundings around the Rh(III) center preventing the approaching of the other assisting molecules. Based on these mechanistic insights, syn-β -OH elimination has also been realized by using Cp*Rh(OAc) 2 as the catalyst affording the enantiomer from the same starting materials. Further studies are currently underway in our laboratory. General method for the Rh-catalyzed β -OH elimination for allene formation reaction is provided in the following To an oven-dried Schlenk tube (25 mL) was added phenylboronic acid 2a (48.9 mg, 0.4 mmol), which was then transferred to a glovebox. After adding [Rh(COD)OH] 2 (2.4 mg, 0.005 mmol) in the glovebox, it was transferred out of the glovebox. After replacing nitrogen with argon for three times by vaccum, ( S )- 1a (40.3 mg, 0.2 mmol, 99% ee) and freshly distilled dioxane (1 mL) were added. The resulting mixture was vigorously stirred at rt for 5 h as monitored by TLC, diluted with ethyl acetate (1 mL), filtered through a short column of silica gel (1 cm), eluted with ethyl acetate (5 mL), and concentrated. 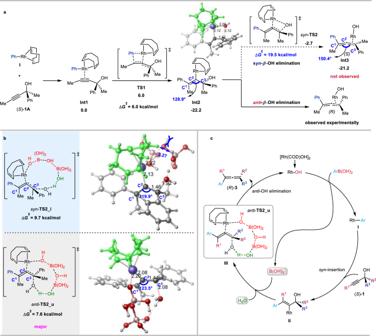Fig. 4: DFT calculations and proposed mechanism for the reaction of (S)-2-phenylpent-3-yn-2-ol (S)-1A with phenyl-rhodium I. aEnergy profiles for thesyn-insertion and the directβ-OH elimination processes of (S)-1Awith phenyl-rhodiumI(Free energies are given in kcal/mol with respect ofInt1).bThe transition states for B(OH)3and H2O assistedanti-β-OH elimination process (Bond lengths are given in angstroms).cThe proposed mechanism. 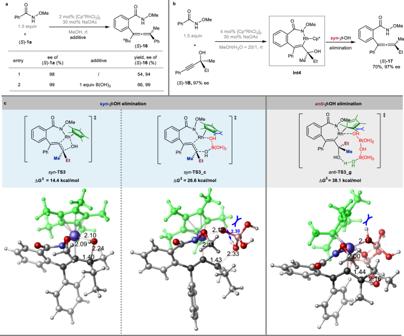Fig. 5: Control experiments and DFT calculations for [Cp*RhCl2]2catalyzed reaction of chiral propargylic alcohol (S)-1B withN-methoxybenzamide45. aControl experiments with or without boric acid.b[Cp*RhCl2]2catalyzed reaction of chiral propargylic alcohol (S)-1BwithN-methoxybenzamide affording chiral allene (S)-17viasyn-β-OH elimination ofInt 4.cThe transition states forsyn- oranti-β-OH elimination process (Bond lengths are given in angstroms). 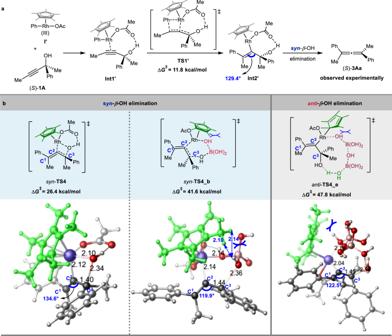Fig. 6: DFT calculations on Cp*Rh(OAc)2catalyzedsyn-β-OH elimination of (S)-2-phenylpent-3-yn-2-ol (S)-1A with Cp*PhRh(III)(OAc) I’. aEnergy profiles for reaction of (S)-1Awith Cp*PhRh(OAc) involving thesyn-insertion andsyn-β-OH elimination process ofInt 2’(Free energies are given in kcal/mol).bThe transition states forsyn- oranti-β-OH elimination process (Bond lengths are given in angstroms). 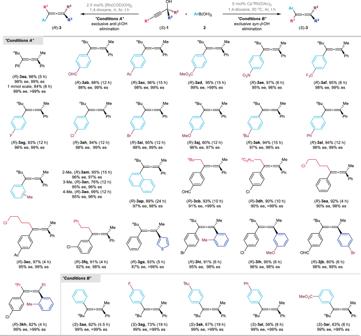Fig. 7: The substrate scope. Conditions A for exclusiveanti-β-OH elimination: (S)-1(0.2 mmol),2(0.4 mmol), and [Rh(COD)OH]2(2.5 mol%) in 1,4-dioxane (1 mL) at rt. Conditions B for exclusivesyn-β-OH elimination: (S)-1(0.2 mmol),2(0.6 mmol), and Cp*Rh(OAc)2(5 mol%) in 1,4-dioxane (1 mL) at 50°C. 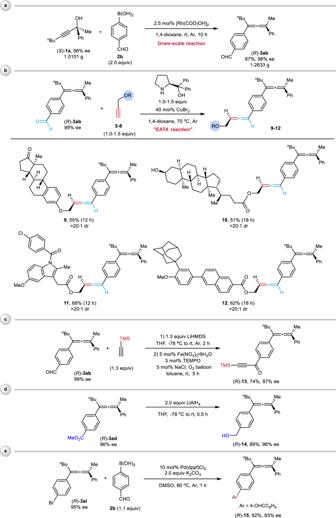Fig. 8: Gram-scale reaction and synthetic transformations of the products. aGram-scale reaction.bCopper-catalyzed enantioselective allenation of (R)-3abwith terminal propargylic ethers5–8.cSynthesis of alkynyl ketone (R)-13from (R)-3ab.dReduction of (R)-3adto alcohol (R)-14with LiAlH4.eSuzuki coupling reaction of (R)-3aito (R)-15with2b. The residue was purified by chromatography on silica gel to afford ( R )- 3aa (51.4 mg, 98%) [eluent: petroleum ether/ethyl acetate = 60/1 (~120 mL)]: 98% ee (HPLC conditions: OJ-H column, hexane/ i -PrOH = 99.5/0.5, 0.7 mL/min, λ = 214 nm, t R (major) = 6.3 min, t R (minor) = 8.0 min); [ α ] D 27 = -326.1 ( c = 1.17, CHCl 3 ); oil; 1 H NMR (400 MHz, CDCl 3 ): δ = 7.43 (t, J = 7.2 Hz, 4 H, Ar-H), 7.29 (m, 4 H, Ar-H), 7.23–7.12 (m, 2 H, Ar-H), 2.62–2.47 (m, 2 H, CH 2 ), 2.20 (s, 3 H, CH 3 ), 1.64–1.49 (m, 2 H, CH 2 ), 1.49-1.35 (m, 2 H, CH 2 ), 0.90 (t, J = 7.4 Hz, 3 H, CH 3 ); 13 C NMR (100 MHz, CDCl 3 ): δ = 205.5, 137.2, 137.0, 128.41, 128.37, 126.7, 126.6, 126.0, 125.6, 107.8, 103.6, 30.1, 30.0, 22.6, 16.8, 14.0; IR (neat): v = 3058, 2954, 2925, 2858, 1932, 1596, 1491, 1443, 1025 cm -1 ; MS (70 eV, EI) m/z (%): 263 (M + + 1, 1.21), 262 (M + , 5.56), 205 (100); HRMS calcd for C 20 H 22 [M + ]: 262.1716, found: 262.1725.